Exercise at depth alters bradycardia and incidence of cardiac anomalies in deep-diving marine mammals Unlike their terrestrial ancestors, marine mammals routinely confront extreme physiological and physical challenges while breath-holding and pursuing prey at depth. To determine how cetaceans and pinnipeds accomplish deep-sea chases, we deployed animal-borne instruments that recorded high-resolution electrocardiograms, behaviour and flipper accelerations of bottlenose dolphins ( Tursiops truncatus ) and Weddell seals ( Leptonychotes weddellii ) diving from the surface to >200 m. Here we report that both exercise and depth alter the bradycardia associated with the dive response, with the greatest impacts at depths inducing lung collapse. Unexpectedly, cardiac arrhythmias occurred in >73% of deep, aerobic dives, which we attribute to the interplay between sympathetic and parasympathetic drivers for exercise and diving, respectively. Such marked cardiac variability alters the common view of a stereotypic ‘dive reflex’ in diving mammals. It also suggests the persistence of ancestral terrestrial traits in cardiac function that may help explain the unique sensitivity of some deep-diving marine mammals to anthropogenic disturbances. Foraging by large, predatory mammals represents one of the most labour-intensive, energetically costly and risky of life-history processes [1] . This is especially apparent for marine mammals, a group that must locate, chase, kill and consume prey while breath-holding and withstanding extraordinary hydrostatic pressures at depth [2] , [3] , [4] . Potential foraging sites for marine mammals range from a few metres below the water surface for sea otters ( Enhydra lutris ) to nearly 3,000 m deep for the Cuvier’s beaked whale ( Ziphius cavirostris ), an extreme diver that is capable of breath-holds longer than 2 h and exposure to pressures exceeding 250 atm (ref. 5 ). Such physiological and physical demands appear incompatible with the exertion required for capturing mobile prey at depth. As a result, the potential for conflict between diving and exercise responses for air-breathing marine predators has remained a long-standing debate [6] , [7] , [8] . The expectation is that marine mammals are adapted for underwater exercise, and thereby uniquely safeguarded from submersion-related injuries that occur in terrestrial species [9] . Presumably, this occurs through a dive response that entails marked reduction in heart rate (bradycardia) and peripheral vasoconstriction during apnoea to conserve limited oxygen reserves [2] , [3] , [4] . However, the impact of exercise on these mechanisms has been difficult to examine in free-ranging marine mammals, particularly cetaceans. In this study, we developed an animal-borne, electrocardiograph-accelerometer (ECG-ACC) depth monitor that provided high-resolution, simultaneous recordings of heart rate (HR), swimming stroke frequency (SF), depth and time throughout the dive ( Supplementary Figs 1 and 2 ). Using a comparative approach, we deployed the instruments on two marine mammal species representing separate evolutionary lineages (pinnipeds and cetaceans) to evaluate the breadth of diving responses among mammals that are adapted for underwater activity. The ECG-ACC was deployed on adult bottlenose dolphins and Weddell seals, and provided detailed behavioural and physiological responses of the animals throughout each dive. Data were recorded for 74 dives from 10 instrumented dolphins trained to dive and exercise at different intensities in pools or open water ranging in depth from the surface to 210 m. The same variables were measured for 91 dives (41 foraging and 50 non-foraging) ranging in maximum depth from 34 to 390 m by three, free-ranging Weddell seals swimming under shore-fast ice in McMurdo Sound, Antarctica during the austral spring. With the exception of dives exceeding 150 m by dolphins, only aerobic dives (that is, those within the aerobic diving limit predicted for each species [2] , [3] , [4] ) were analysed in this study. Here we report that dive depth and exercise level alter the intensity of bradycardia associated with the dive response, which in turn, impacted the incidence of cardiac anomalies observed for two evolutionarily distinct lineages of marine mammals. Specifically, we show that the frequency of cardiac arrhythmias increases with elevated SFs and becomes more pronounced in deeper dives. Such cardiac variability during diving challenges the current understanding of adaptive safeguards in marine mammals, and may provide an important link between behaviour and susceptibility to diving injuries in this group. 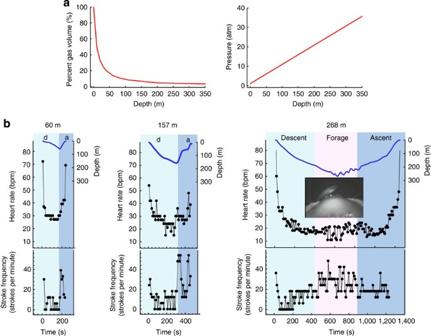Figure 1: Physical and physiological changes with dive depth in Weddell seals. (a) Changes in gas volume (as in the lung11, left) and hydrostatic pressure19(right) with dive depth are compared. (b) HR and corresponding SF in relation to dive time for shallow (left), mid-range (middle) and deep-foraging dives (right) by a Weddell seal. Depth is denoted by the top blue line. Circles represent 10 s HR and SF analysis intervals. Descent (d) and ascent (a) periods are indicated by light blue and dark blue backgrounds, respectively. The effect of silverfish captures (pink area) was confirmed by ‘over-the-nose’ video recordings (inset). Note the progressive decrease in minimum HR with depth from 27 bpm for the 60 m dive, then 15 bpm for 157 m to 10.8 bpm for the 268 m dive. Bradycardia varies with depth and exercise in diving mammals Behaviourally linked ECGs of freely diving Antarctic seals and trained dolphins ( Table 1 ) revealed a complex dive response that was altered by several integrative factors. Instead of a single level of bradycardia, HR while submerged varied with both depth ( Fig. 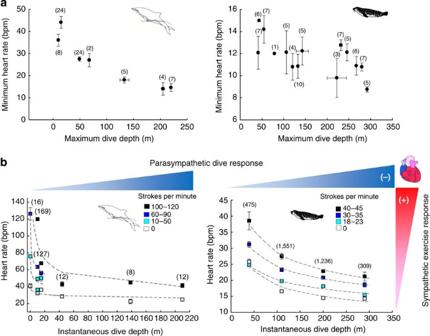Figure 2: HR in relation to maximum and instantaneous dive depth for bottlenose dolphins and Weddell seals. (a) Minimum HR is plotted in relation to maximum dive depth, with number of dives indicated in parentheses. (b) Symbols representing mean HR at instantaneous depths include data for maximum and transit depths during ascent and descent; values are colour-coded for exercise intensity based on SF (insets). Dashed lines are the least squares power regressions (P<0.0005). Numbers in parentheses show the total number of HR intervals measured for each depth. Bordering triangles denote hypothetical grade changes in parasympathetic diving response (blue) and sympathetic exercise response (red) representing the major neural drivers for HR. Symbols and vertical or horizontal lines show mean±1 s.e.m. (Note that SFs for dolphins diving >100 m are based on levels measured for animals wearing video cameras39). 1 and Table 2 ) and exercise intensity ( Fig. 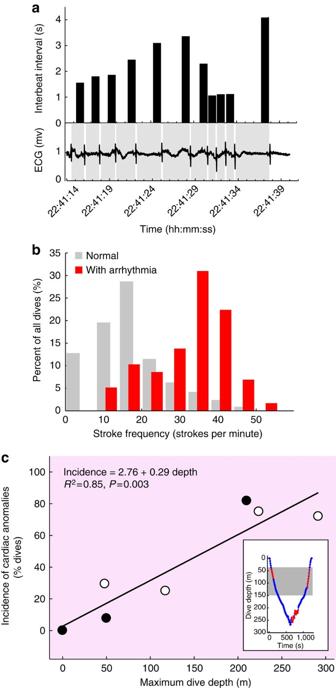Figure 3: Cardiac anomalies in diving seals and dolphins. (a) Rapid changes in the ECG trace (bottom) in real time for a submerged swimming seal corresponded to marked fluctuations in inter-beat interval (IBI, top). Vertical lines in the ECG denote the QRS complex and individual heart beats. Grey bars indicate the r-r interval on which IBI (black bars) is based. (b) Percentage distribution of SFs used by seals throughout normal dives (grey bars) and during arrhythmic cardiac events (red bars,n=91 dives). (c) Percentage of dives displaying cardiac anomalies in relation to maximum dive depth for dolphins (black symbols,n=26 dives) and seals (white circles,n=90 dives). The solid line is the least squares linear regression as described in the figure. The inset illustrates a typical time-depth profile for a seal with normal (blue) and arrhythmic (red) periods indicated. The grey box denotes depths associated with lung collapse/expansion10,11,12. 2 and Table 3 ). The change in HR with depth was nonlinear, following patterns for gas volume changes that occur with increasing hydrostatic pressure at depth ( Fig. 1a ). Indeed, the greatest change (69% and 88% for seals and dolphins, respectively) in HR during a dive occurred between the water surface and depths (ca. 100–150 m) typically associated with rapid lung compression (descent) or expansion (ascent) [10] , [11] , [12] . HR declined asymptotically with instantaneous dive depth (that is, location in the water column), reaching a minimum as the animals descended to the dive bottom ( Fig. 1b ). Both species showed a negative correlation between minimum HR and maximum dive depth ( Fig. 2a ). Table 1 Morphometrics, study location and instrumentation used on bottlenose dolphins and Weddell seals in this study. Full size table Figure 1: Physical and physiological changes with dive depth in Weddell seals. ( a ) Changes in gas volume (as in the lung [11] , left) and hydrostatic pressure [19] (right) with dive depth are compared. ( b ) HR and corresponding SF in relation to dive time for shallow (left), mid-range (middle) and deep-foraging dives (right) by a Weddell seal. Depth is denoted by the top blue line. Circles represent 10 s HR and SF analysis intervals. Descent (d) and ascent (a) periods are indicated by light blue and dark blue backgrounds, respectively. The effect of silverfish captures (pink area) was confirmed by ‘over-the-nose’ video recordings (inset). Note the progressive decrease in minimum HR with depth from 27 bpm for the 60 m dive, then 15 bpm for 157 m to 10.8 bpm for the 268 m dive. Full size image Table 2 Regression statistics for heart rate in relation to depth for diving dolphins and seals. Full size table Figure 2: HR in relation to maximum and instantaneous dive depth for bottlenose dolphins and Weddell seals. ( a ) Minimum HR is plotted in relation to maximum dive depth, with number of dives indicated in parentheses. ( b ) Symbols representing mean HR at instantaneous depths include data for maximum and transit depths during ascent and descent; values are colour-coded for exercise intensity based on SF (insets). Dashed lines are the least squares power regressions ( P <0.0005). Numbers in parentheses show the total number of HR intervals measured for each depth. Bordering triangles denote hypothetical grade changes in parasympathetic diving response (blue) and sympathetic exercise response (red) representing the major neural drivers for HR. Symbols and vertical or horizontal lines show mean±1 s.e.m. (Note that SFs for dolphins diving >100 m are based on levels measured for animals wearing video cameras [39] ). Full size image Table 3 Regression statistics for heart rate in relation to stroke frequency for diving dolphins and seals. Full size table Superimposed on this depth response was an increase in HR that varied with the level of physical exertion ( Fig. 2b and Table 3 ). For all depths, HR was lowest when animals were resting, gliding or exhibiting low activity levels typical of routine swim speeds. When SF was equal to 0 (at rest or gliding), the relationship between HR and depth was described as follows: for dolphins, and for seals, where HR is in beats per minute and depth is in metres. As evident from the increase in the coefficients, these relationships were shifted upwards as SF increased in accordance with species-specific performance and depth ranges. 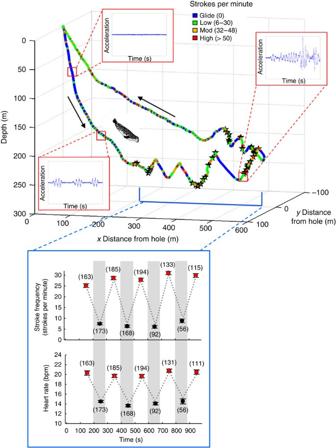Figure 4: Behavioural control of exercise intensity and HR by foraging seals. A typical three-dimensional dive plot shows depth in relation to distance from a breathing hole as colour-coded for SF. Black stars denote silverfish captures during the saw-tooth segment. Insets are the corresponding traces from the ACC illustrating the three primary swimming behaviours—gliding (blue), stroke-and-glide (intermittent blue and green), and constant, high-amplitude stroking before and during fish capture and initial ascent (green to orange to red). Each point represents 1 s. The lower panel illustrates sequential cardiac and kinematic changes in relation to time during descent (black circles, grey bars) and ascent (red circles) of the saw-tooth dive segment (n=41, foraging dives). Circle and whiskers are mean±1 s.e.m. Numbers in parentheses represent the number of data points for all dives. Bottlenose dolphins, a comparatively shallow diving species [13] , showed a 1.7–3.7-fold increase in HR over gliding values during the highest level of exercise (100–120 strokes per minute) as described by Weddell seals, a deep-diving specialist [2] , [4] , showed a 1.5–1.8-fold increase in HR over gliding values at the highest exercise level (40–45 strokes per minute) according to the equation given below: HRs of diving seals integrate multiple factors A general linear model indicated that depth, SF, and body size were significant factors that set the HR of the deep-diving seals ( n =7,283 matched HR intervals; P value <0.0005), but that the interaction term between SF and depth was not ( Table 4 ). Whether body mass per se or other factors (for example, behaviour) associated with size also affected HR could not be determined. Importantly, because each data point for the dolphins and seals is based on instantaneous depth, each includes HR values for descent, bottom and ascent segments of dives. Thus, depth of the animal rather than simply dive duration appears to be an important modifier of the exercise response ( Table 3 ). Table 4 Regression statistics for two- and three-factor general linear models relating heart rate to depth, stroke frequency and body mass in three Weddell seals. Full size table Cardiac arrhythmias occur in deep divers Rather than a graded, stable bradycardia at depth, Weddell seals displayed irregular patterns in inter-beat interval (IBI) that were characterized by brief, alternating periods of tachycardia and bradycardia ( Fig. 3a ). Independent ectopic heart beats ( Supplementary Fig. 2 ) were often evident during these periods, particularly during constant elevated SF ( Fig. 3b ) as during initial ascent from deep dives. The resulting mean stroking rate for normal (16.4±10.2 strokes per minute, range=0–54 strokes per minute, n =7,917) and arrhythmic (34.4±9.8 strokes per minute, range=12–54 strokes per minute, n =53) periods differed significantly ( t =10.81, P value <0.0005, df=52, Student’s t -test; Fig. 3b ). Figure 3: Cardiac anomalies in diving seals and dolphins. ( a ) Rapid changes in the ECG trace (bottom) in real time for a submerged swimming seal corresponded to marked fluctuations in inter-beat interval (IBI, top). Vertical lines in the ECG denote the QRS complex and individual heart beats. Grey bars indicate the r-r interval on which IBI (black bars) is based. ( b ) Percentage distribution of SFs used by seals throughout normal dives (grey bars) and during arrhythmic cardiac events (red bars, n =91 dives). ( c ) Percentage of dives displaying cardiac anomalies in relation to maximum dive depth for dolphins (black symbols, n =26 dives) and seals (white circles, n =90 dives). The solid line is the least squares linear regression as described in the figure. The inset illustrates a typical time-depth profile for a seal with normal (blue) and arrhythmic (red) periods indicated. The grey box denotes depths associated with lung collapse/expansion [10] , [11] , [12] . Full size image We attribute these HR patterns to the interplay between contrasting sympathetic and parasympathetic neural drivers that control the mammalian heart [14] , [15] . Sympathetic stimulation that occurs with exercise promotes an increase in HR (tachycardia), while increased parasympathetic stimulation mediates slowing of the heart (bradycardia) during the dive response by marine mammals [16] , [17] , [18] . A graded increase in parasympathetic stimulation coinciding with changes in instantaneous depth would explain the progressive decline in HR with depth at each exercise level ( Fig. 2b ), and is consistent with the dampening effect on HR observed for harbour seals voluntarily diving in pools [17] . Under the free-ranging conditions examined here, this graded neural drive also explains the gradual development of bradycardia during initial descent, even while the animals are gliding to depth and at near-resting metabolic rates. The physiological mechanism underlying a graded depth response is currently unknown, but is likely integrative. At the level of myocardial cells, hydrostatic pressure can modify both beat frequency (chronotropic function) and contraction force (inotropic function) of the heart [19] . Baroreceptors [20] , pulmonary stretch receptors [21] , blood gases [4] , cardiovascular hormones (for example, natriuretic peptides) [22] , [23] as well as physical changes in lung volume and pulmonary shunting with the rise and fall of hydrostatic pressures during descent and ascent influence HR in diving humans and marine mammals [15] , [18] . The well-documented, progressive collapse and re-inflation of the lungs of diving dolphins [10] , [11] and pinnipeds [2] , [12] as the animals pass 40–150 m would also support a graded hydrostatic mechanism affecting HR [21] ( Fig. 1a ). Regardless of the underlying mechanisms, normal cardiac rhythms can be disrupted when cardiac-stimulating and cardiac-suppressing neural signals switch quickly [24] . In human breath-hold divers, when exercise is superimposed on the diving response, sympathetic neural activation dictates cardiac variability and the ultimate level of bradycardia that is achieved [25] , [26] . Similarly, in deep-diving Weddell seals, IBI fluctuated rapidly between short periods of tachycardia and bradycardia, especially during dive ascents ( Fig. 3a ). Similar to humans [24] , [25] , [26] , these irregular IBI patterns were associated with independent ectopic heart beats that were most evident during periods of constant elevated SF ( Fig. 3b ). Theoretically, the greatest disparity between exercise- and dive-related neural drivers for HR, and thus the greatest potential for arrhythmia events, will occur during the highest SFs at the deepest depths. Such was observed for the animals in this study ( Fig. 3b,c ). For dolphins, >81% of dives to 210 m ( n =11) showed high levels of cardiac variability and arrhythmic periods (as determined from sequential changes in mean HR; see Methods section below) during directed ascent compared with only 7.7% of dives to 60 m ( n =13; Fig. 3c ). Likewise, only 26.3% of shallow dives at <100 m ( n =19) by Weddell seals included arrhythmias while 73.1% of deep dives (mean=289.7±7.9 m, n =26) displayed some form of cardiac anomaly. The majority (67.3%) of cardiac arrhythmias during deep dives by seals occurred during continuous stroking associated with ascent including the initial turnaround from maximum depth and then the final ascent to the surface at 45–116 m (mean=78.2±7.3 m). It is noteworthy that mean arrhythmia depth on descent (58.5±7.6 m, n =20) and final ascent occurred within the purported range of depths associated with lung collapse/re-inflation owing to changing hydrostatic pressures [2] , [10] , [11] , [12] ( Fig. 3c , inset). Cardiac variability during submergence is not unique to the species in this study and has been reported for human breath-hold divers [26] , [27] , grey seals ( Halichoerus grypus [28] ) and California sea lions ( Zalophus californianus [29] ). In submerged humans [24] , [30] , as for Weddell seals ( Fig. 3a ), cardiac arrhythmias often occur in association with alternating short periods of tachycardia and bradycardia correlated with exercise. Based on this, it is not surprising that the swimming segment of cold water triathlons accounts for over 90% of race day deaths in human athletes [31] with cardiac malfunction cited as an underlying contributing factor [24] . For dolphins and the three pinniped species noted above, ectopic heart beats were most apparent during ascents from the deepest foraging dives [28] , [29] ( Fig. 3c ). What is surprising from our study is the frequency of occurrence of these cardiac anomalies and the similarity of the response to those of submerged terrestrial mammals by two different evolutionary lineages of marine mammals that are otherwise adapted for underwater activity. Our study shows that 50 million years of physiological evolution along the land-to-sea transition of marine mammals [32] may not have completely solved the problem of balancing cardiac responses for underwater exercise. Rather, the results suggest that the primary adaptation for diving by marine mammals supports normal cardiac function during species-specific routine dive depths. But this adaptation is limited, as evident from the rise in cardiac anomalies with increased physical exertion during ascent from the deepest dives ( Fig. 3c ). For foraging marine mammals, precise linking of swimming behaviours to specific dive segments ( Supplementary Videos 1 and 2 ) when chasing prey facilitates cardiac stability, ostensibly by diminishing the potential for rapid changes in opposing exercise and diving responses controlling HR. We found that foraging Weddell seals preferentially used low intensity swimming modes (gliding and low stroke amplitude burst-and-glide swimming) on initial descent ( Fig. 4 ). Like other pelagic marine mammals, including humpback whales ( Megaptera novaeangliae [33] ), the seals changed to a relatively horizontal saw-tooth pattern of gliding descents and short ascending prey chases within 25.4±0.7% of maximum dive depth ( n =666 fish encounters) when feeding on Antarctic silverfish ( Pleuragramma antarcticum ). Alternating periods of low (10.3±0.3 strokes per minute, n =827) then moderate (28.3±0.4 strokes per minute, n =789) exercise levels for each descent and ascent segment of the saw-tooth were reflected in predictable, alternating low (15.1±0.1 bpm, n =826) then modest increases (20.1±0.2 bpm, n =745) in HR ( Fig. 4 ). The most common trigger for cardiac arrhythmias, high amplitude high SF (>30 strokes per minute), occurred primarily during the initial ascent and was quickly replaced by burst-and-glide swimming to the surface ( Fig. 4 ). Figure 4: Behavioural control of exercise intensity and HR by foraging seals. A typical three-dimensional dive plot shows depth in relation to distance from a breathing hole as colour-coded for SF. Black stars denote silverfish captures during the saw-tooth segment. Insets are the corresponding traces from the ACC illustrating the three primary swimming behaviours—gliding (blue), stroke-and-glide (intermittent blue and green), and constant, high-amplitude stroking before and during fish capture and initial ascent (green to orange to red). Each point represents 1 s. The lower panel illustrates sequential cardiac and kinematic changes in relation to time during descent (black circles, grey bars) and ascent (red circles) of the saw-tooth dive segment ( n =41, foraging dives). Circle and whiskers are mean±1 s.e.m. Numbers in parentheses represent the number of data points for all dives. Full size image Behavioural control of exercise at depth, as demonstrated here, enables marine mammals to perform deep-sea chases within the physiological limits imposed by the mammalian cardio-respiratory system. In view of this, are there consequences when routine behaviours are disrupted? We have found that behaviours contributing to cardiac anomalies when submerged (elevated levels of physical exertion, deep-diving and rapid ascent from depth) are remarkably similar for terrestrial [18] , [24] , [25] , [26] , [27] and marine ( Figs 1 , 2 , 3 , 4 ) mammals. Coincidentally, these also comprise the suite of behaviours displayed during the flight response of beaked whales [34] and blue whales [35] exposed to shipping noise and mid-frequency sonars. Admittedly, the physiological repercussions of the flight responses are currently unknown. However, these responses have the potential to override behavioural safeguards that maximize cardiac stability in extreme divers ( Fig. 4 ), and warrant consideration when assessing possible impacts of man-made disturbances on oceanic mammals. Experimental approach We instrumented trained bottlenose dolphins and wild Weddell seals with submersible ECG-ACC monitors ( Table 1 ). Video recorders [36] and two- to three-axis accelerometers with pressure meters incorporated into the instruments were used to simultaneously monitor swimming SF and depth throughout the dives. The combination of instruments allowed us to precisely match instantaneous cardiac responses to swimming biomechanics, activity level, underwater behaviour, depth and prey capture events ( Supplementary Video 1 ). Animals Ten adult bottlenose dolphins ( Tursiops truncatus ) and three adult male Weddell seals ( Leptonychotes weddellii ) were used in the HR studies. Five male dolphins were housed in saltwater pools ranging from 3 m in depth at Long Marine Laboratory (University of California, Santa Cruz) to 10 m deep at Disney’s Epcot The Seas exhibit (Lake Buena Vista, FL). Three dolphins (two males and 1 female) were housed at the Dolphin Experience (Freeport, Grand Bahamas Island) in large (15 m × 15 m × 5 m deep) pens connected to the open ocean. Data collected previously from two additional dolphins housed in saltwater pens in Oahu, HI [37] were analysed and included (see ‘HR variability in deep-diving dolphins’ section below). All dolphins were fed multiple times daily on a mixed fish diet (mackerel, herring, squid and capelin depending on facility) supplemented with vitamins. Water temperature, in the pools was 20.0–25.0 °C and ocean temperature ranged from 23.5 to 25.0 °C during the test period. Weddell seals were captured in McMurdo Sound near Ross Island, Antarctica during the winter and austral spring 2009–2010. The methods for capturing, attaching animal-borne instruments and recovering the instruments on free-ranging Weddell seals has been described previously [36] . In brief, adult seals were approached on the sea ice, captured in a purse seine net and transported to a hut located within 7–11 km of the capture point. Following sedation and weighing, the instruments were attached to neoprene patches glued onto the back and head of the animals. The complete instrument package included the ECG-ACC microprocessor described below and a miniaturized video data acquisition platform [36] . After an overnight recovery, the animals were released into a nearby ice hole and were free to dive and forage for ~5–21 days at which point the seals were recaptured and instrumentation was removed for data download and analysis. All animal procedures were conducted under National Marine Fisheries Service OPR permits to T.M.W. and were approved by each facility's Institutional Animal Care and Use Committee with the UCSC committee as oversight. Sample size for animals used in this study was determined by power analyses for physiological responses coupled with animal availability and level of training (dolphins). Study design Dolphins were studied under three experimental conditions as follows: (1) voluntary rest on the water surface, (2) rest while submerged, and (3) during submerged swimming and diving exercise. Resting measurements were taken while the animals floated dorsal side up next to a dock or as they stationed in front of a trainer at depth. Exercise tests consisted of a descent, horizontal steady-state swimming through a series of submerged hoops positioned on the bottom of a saltwater pool (Epcot) or along the sandy bottom of a dive (Bahamas) followed by ascent. Each animal selected preferred ‘slow’, ‘moderate’ and ‘fast’ speeds, as well as diving duration. A trained sprint ascent from 15 m to the surface was also evaluated for the open water dolphins. All dolphins were trained over at least 6 months using positive operant conditioning to swim at various speeds before data collection. Each experimental session lasted ~15 min and began with 1–5 min of surface resting following instrumentation. Individual dives were then randomly divided into submerged resting or swimming trials. Physiological data for Weddell seals were recorded as the animals freely moved throughout McMurdo Sound. Both foraging and non-foraging dives (confirmed from capture events on accompanying videos) were evaluated. Maximum depth was dependent on location in the Sound and reached ~390 m for the dives used in the present analysis. ECG waveforms, swimming SF, depth and behaviour were recorded simultaneously during resting periods and dives for both species, providing unprecedented detail of kinematic, behavioural and physiological events at depth ( Supplementary Videos 1 and 2 ). Video recordings (seals and dolphins) and observers with stopwatches (dolphins only) synched to the internal clock of the instruments maintained a running diary of the duration and type of all underwater events. HR and SF To circumvent potential interference of skeletal muscle noise on cardiac events, we recorded entire ECG waveforms rather than HR per se during the dives. We designed two submersible ECG units for these studies. The first unit, an IQmark Advanced Holter (version 7.2) ECG monitor (Midmark Diagnostics Group, Versailles, OH) placed in a waterproof housing (18 cm × 8 cm × 4.5 cm; Backscatter Underwater and Video, Monterey, CA) was only used on dolphins. A second smaller (16 cm long × 3 cm diameter tube) custom-designed HR unit (ECG-ACC depth recorder; UUB/4-EIAP ECG/IBI/Acceleration/Pressure Recording System, UFI, Morro Bay, CA) used on dolphins and seals simultaneously recorded ECG, SF from either a two- or a three-axis accelerometer, and hydrostatic pressure that was converted to water depth. Signals from each transducer were recorded at 50–100 Hz. To record ECGs, two suction cup electrodes (5 cm diameter with a 2-cm diameter silver plate electrode) were placed on the sternum of the dolphins directly below the pectoral fin insertions, and above the right scapula according to Noren et al . [8] For the Weddell seals, two 2 cm diameter silver electrodes were placed on shaved areas of skin in lateral and ventral axillary areas, and covered with neoprene patches glued to the fur. Shielded wires soldered to the electrodes were connected to the monitors and enabled ECG waveforms to be recorded continuously throughout the experimental sessions ( Supplementary Fig. 1 ). Accuracy of the monitors and electrodes was tested immediately before deployment by simultaneously using a Polar HR watch or a UFI Simple Scope ECG signal display monitor (SC-2000, UFI). Muscle noise from hind flipper movements was generally in the form of a baseline deformation that could be corrected and did not interfere with the IBI analyses (see section ‘Defining arrhythmias’ below). With extreme activity when the fore flippers, head and neck were moving (as during fish consumption), muscle noise was evident and could be used to confirm fish captures ( Supplementary Video 1 ). Any trace in which the ECG waveform was not evident, the segment of the dive or the entire dive was omitted from the data set. For the bottlenose dolphins, the submersible ECG-ACC recorder was attached to a custom-sized neoprene rubber vest (O’Neill, Santa Cruz, CA) that was fitted around the chest of the animal. For seals, the recorders were placed in a neoprene pocket attached to a neoprene patch glued directly onto the fur along the dorsal midline. Size of the instrumentation represented <5% of the frontal area of the animals. Previous tests with larger profile units have demonstrated little (<10%) or no change in speed, stroke mechanics or energetic cost to instrumented marine mammals [38] . Defining arrhythmias The definitive QRS complex from each ECG waveform allowed fine resolution detection of ectopic beats as well as changes in IBIs (defined below under the section ‘Analysis and statistics’); these represented the most prevalent cardiac anomalies in the diving seals and dolphins. Although there was evidence of wandering pacemakers, and rarely, pre-ventricular contractions, we could not discount individual variation in blubber thickness and the non-human clinical placement of the electrodes as factors in waveform shape. Thus, to remain conservative, we report only definitive arrhythmia results (that is, ectopic beats and irregular IBI patterns) and state that these represent an unsteady ‘cardiac state’ rather than a lethal physiological condition. Individual ectopic beats were identified as IBI <1.6 s, which represents values outside of the normal range of average HR responses during diving, and/or a >60% increase in HR from the previous beat coupled with a >30% decline in HR in the subsequent beat ( Supplementary Fig. 2 ). Using this definition, we were able to identify individual cardiac anomalies as opposed to simple adjustments in HR that may occur over several sequential beats. HR variability in deep-diving dolphins In addition to detailed ECG recordings for shallow diving dolphins, we examined the effects of deep dives on variability in HR in two adult female bottlenose dolphins trained to dive to 60, 150 and 210 m in open water off the coast of Oahu, HI. Methods have been reported previously [37] . In brief, dolphins were transported by boat to dive sites, were released and trained to dive in a straight-line path to a submerged buoy. HR and depth were monitored continuously with a waterproof microprocessor (2.5 cm diameter × 15 cm long; Wildlife Computers, Inc., Redmond, WA) and recorded as running means over 10 and 1 s, respectively. Instrumentation and two cross-chest electrodes connected to the microprocessor were incorporated into a low-profile nylon harness worn by the diving dolphins. All dives ≤150 m in depth were within the aerobic dive limit of the dolphins as determined previously from changes in blood lactate concentration [37] . Here we analysed the microprocessor data to assess variability in cardiac responses during prolonged, deep dives. This included HR in relation to maximum dive depth and instantaneous HR during two known SF periods. Because the microprocessor recorded mean HR over 10 s intervals, it was not possible to determine discrete arrhythmia events. Rather, periods of cardiac instability were identified from sequential changes in mean HR and variance calculated from a running average of three successive 10-s intervals throughout the dives. Fluctuations in the means and variance for deep-diving dolphins were compared with similar analyses from detailed ECG recordings for dolphins in the 15-m trials in which no arrhythmias were apparent. Using this baseline, we set a change of ≥36 bpm in sequential mean HR as an indicator of elevated variability. In this way, the analysis accounted for normal progressive changes in HR as well as identified periods of the dive associated with spontaneous spikes in HR. Although SF was not monitored during the HR trials with deep-diving dolphins, we have previously reported two characteristic periods of known SF using animal-borne video cameras for the same-sized, trained dolphins performing these deep target dives ( Supplementary Video 2 and refs 13 , 39 ). These highly trained animals performed a stereotypical pattern of behaviours to complete the deep dives. This included gliding at the bottom of the descent as the underwater buoy was reached and high-frequency, high-amplitude stroking on initial ascent (confirmed by scuba diver observation and mounted cameras for dives <50 m, and animal-borne cameras at deeper depths). During these periods, swimming SF was 0 and 110 strokes per minute, respectively. By presenting the SF data for dolphins in categorical form, we are confident that the minimum and maximum performance levels reported here are represented appropriately in this study. Analysis and statistics For each session, ECG-ACC outputs and depth were recorded continuously. The number of heart beats (r–r intervals) and corresponding swimming stroke cycles were manually counted using UFI software imported to Excel (Microsoft Office, 2010) at 5–10 s (dolphins) and 10 s (seals) periods for the entire dive record. Sequential IBIs were initially detected and analysed using an automated IBI algorithm (UFI, Morro Bay, CA). This was verified by manual calculation of r-r intervals for each heart beat within segments of the time-stamped ECG trace containing arrhythmias. In contrast to previous analyses [7] , [8] , transition periods during ascent and descent were examined in addition to the steady-state exercise responses while swimming at depth. To make the data sets comparable between species, we limited the ECG analyses to dives that remained within reported species-specific calculated aerobic dive limits [2] , [3] , [4] . Because the purpose of this study was to evaluate the inter-relationships between HR, SF and depth, we first determined the ECG analysis interval that (1) surpassed the potential lag period between HR responses and SF, and (2) provided the greatest distinction between depths. For trained dolphins performing shallow (<20 m) dives, a 5-s analysis interval was used owing to the short transit time to depth; the analysis interval was increased to 10 s for deeper dives. Trained dolphins performed swimming tests at specific depths to simulate foraging activities, and the resulting data were categorized according to each trial depth. For free-ranging Weddell seals where performance depth was selected by the animal, each dive was divided into four categories representing shallow depths (<50 m), mid-range depths below the estimated point of lung collapse (35–150 m; refs 2 , 12 ) and deep-foraging depths (155–250 m and >250 m) as determined from known dive behaviours and classifications [40] . The minimum ECG analysis interval was determined by evaluating the sequential changes in seal HR during glide sequences where SF levels remained constant. Mean HR was determined for progressively longer intervals from 5 to 30 s. Differences between pre-glide and interval means for HR were determined by t -tests (Sigma Stat 3.5-SYSTAT, Jandel Scientific, 2005). The results showed that an ECG analysis interval of 10 s for Weddell seals satisfied the study criteria (at P value <0.001, Student’s t -test; Supplementary Fig. 3 ). Least squares methods (SYSTAT, 2005) were used to examine the relationship between HR and depth, and HR and SF for each species, depth and exercise category. Data for resting and gliding (where SF=0) were used in the HR–depth analyses for both species and in the HR–SF analysis for the dolphins where rest and glide periods were defined by trainers. When specifically examining the effect of SF on HR for wild seals, SF=0 on a dive could represent (1) inactive on the bottom, (2) inactive in the water column, (3) gliding through the water column, (4) gliding along the bottom or (5) resting on the surface. Because each of these conditions may represent different physiological states and could not be definitely differentiated in all cases for the wild animals, we limited the HR–SF data to actively stroking animals for which the performance level was known. Differences in the resulting regressions of HR on SF between depths were determined from ANCOVA tests using statistical software (SYSTAT, 2005) for n =2 depths for the dolphins and n =4 depths for the seals. These results were compared with HR and SF values reported for surface swimming dolphins chasing a boat at 2.1–2.9 m s −1 ref. 41 and for deep-diving dolphins [37] as described above. Mean values±1 s.e.m. are presented unless otherwise indicated. Two-factor and three-factor general linear models (SYSTAT version 13, 2009) were used to examine the inter-relationships between HR (in beats per minute) and three factors: depth (m), SF (in strokes per minute) and body mass (kg) for the three seals in this study ( Table 4 ). Models were compared using adjusted R 2 , Akaike’s information criterion and by examining residuals for each animal during ascent and descent. Adjusted R 2 and Akaike’s information criterion for each model are presented with the best model shown in bold in Table 4 Similar analyses were not conducted for the dolphins owing to the limited range of depths represented by each animal. Correlations between arrhythmia incidence and instantaneous and maximum dive depths were determined using linear least squares methods (SYSTAT, 2005). Corresponding acceleration patterns from swimming movements were also examined using both UFI and Pro-Analyst (version 1.5.6.5. Cambridge, MA: Xcitex Inc., 2003–2013) software. In this way, potential artefacts associated with muscle noise on arrhythmia detection could be identified. Pro-Analyst software was also used to synchronize video records with ECG and swimming stroke acceleration patterns of the seals. This enabled behavioural events including fish captures and chases at depth to be correlated with cardiac and locomotory responses ( Supplementary Video 1 ). Statistical data reported in this paper are tabulated in Tables 2 and 3 . Additional access to the data may be found through the additional data file and the corresponding author. How to cite this article : Williams, T. M. et al . Exercise at depth alters bradycardia and incidence of cardiac anomalies in deep-diving marine mammals. Nat. Commun. 6:6055 doi: 10.1038/ncomms7055 (2015).